Single-crystal diamond nanomechanical resonators with quality factors exceeding one million Diamond has gained a reputation as a uniquely versatile material, yet one that is intricate to grow and process. Resonating nanostructures made of single-crystal diamond are expected to possess excellent mechanical properties, including high-quality factors and low dissipation. Here we demonstrate batch fabrication and mechanical measurements of single-crystal diamond cantilevers with thickness down to 85 nm, thickness uniformity better than 20 nm and lateral dimensions up to 240 μm. Quality factors exceeding one million are found at room temperature, surpassing those of state-of-the-art single-crystal silicon cantilevers of similar dimensions by roughly an order of magnitude. The corresponding thermal force noise for the best cantilevers is ~5·10 −19 N Hz −1/2 at millikelvin temperatures. Single-crystal diamond could thus directly improve existing force and mass sensors by a simple substitution of resonator material. Presented methods are easily adapted for fabrication of nanoelectromechanical systems, optomechanical resonators or nanophotonic devices that may lead to new applications in classical and quantum science. Nanomechanical resonators have led to pioneering advances in ultrasensitive sensing and precision measurements. Applications range from nanoscale detection of forces in the context of scanning probe microscopy [1] to molecular-recognition-based mass screening in the medical sciences [2] . The sensitivity of submicron-thick devices has progressed to a point where the attonewton force of single spins [3] or the mass of single molecules and proteins [4] , [5] can be measured in real time. Singly clamped cantilever beams have been pivotal in several fundamental physical discoveries, including the detection of persistent currents in normal metal rings [6] and the observation of half-height magnetization steps in Sr 2 RuO 4 (ref. 7 ). Resonators coupled to optical cavities [8] or spins [9] are furthermore intensively explored as quantum mechanical device elements in quantum science and technology. A key figure of merit for a sensitive mechanical resonator is the rate at which it gains or looses mechanical energy, described by the mechanical quality factor Q . In the quantum mechanical regime, for example, the life time of an oscillator’s vibrational ground state is where ω c is the resonator frequency and k B T is the thermal energy. Thermomechanical noise also limits the sensitivity toward measurement of small forces, with a minimum detectable force (per unit bandwidth) given by where k c is the spring constant. State-of-the-art silicon cantilevers can achieve force sensitivities of typically 10 −16 N Hz −1/2 at room temperature and 10 −18 N Hz −1/2 at millikelvin temperatures [10] , [11] . Despite considerable effort, attempts to improve this sensitivity well into the zeptonewton-range (1 zN=10 −21 N) have not been particularly successful. One strategy has been the development of thinner, more compliant resonators with lower spring constant k c ( μ N·m −1 –mN·m −1 ). The projected gain in sensitivity, however, was found to be counteracted by a decrease in the mechanical Q with decreasing thickness due to surface friction [12] , [13] . Several other routes have been explored, including, for example, surface cleaning under ultra high-vacuum conditions [14] or the use of doubly clamped beams at high spring tension [15] . Exciting recent progress has further been made with bottom-up devices such as suspended carbon nanotube [16] , silicon nanowire [17] or trapped ion [18] oscillators. All of these approaches have their drawbacks, however. For example, ultra high-vacuum conditions are often not sustainable, high spring tensions lead to no net gains in force sensitivity (due to increased stiffness) and the geometry of bottom-up devices may not be compatible with many applications. The goal of the current effort is to explore whether single-crystal diamond may serve as a low dissipation material for sensitive nanoelectomechanical systems (NEMS) and microelectomechanical systems (MEMS) applications. As diamond excels in many properties such as mechanical strength, optical transparency, thermal conductivity and chemical resistance, the material is an interesting platform for integrated-nanoscale devices. Diamond is, for example, a promising choice for low-loss photonic devices [19] , [20] and ultra-high-frequency mechanics [21] . In addition, diamond hosts interesting intrinsic dopants—most prominently the nitrogen-vacancy centre—that have been recognized as rich resource for single-photon generation [22] , quantum engineering [23] and nanoscale magnetic sensing [24] . A particularly interesting perspective is the use for optomechanical transducers that exploit all the mechanical, optical and dopant properties offered by the material. Unfortunately, fabrication of single-crystal diamond into high-quality MEMS and NEMS is notoriously difficult, and only over the last few years has material amenable to nanofabrication become available [25] . To illustrate the challenges in fabricating single-crystal diamond nanostructures, one may note that the material cannot be grown on any other substrate than single-crystal diamond itself [25] , precluding wafer-scale processing. Early diamond NEMS have therefore focused on polycrystalline diamond that can be readily grown as a thin film on various substrates, including silicon. In 2004, researchers demonstrated fabrication of 40 nm-thin devices (grain size 10–100 nm) exhibiting Q factors up to 10,000 at cryogenic temperatures [26] , [27] . Only recently have researchers tackled fabrication of single-crystal diamond MEMS and NEMS. In the absence of wafer material, the main route to producing thin films has relied on ion bombardement. In this approach, a flat diamond surface is exposed to a large dose of high energy (MeV) ion irradiation, resulting in a damage layer typically a few hundred nanometres below the surface that can be selectively etched to peel off thin membranes [28] . Impinging ions, however, have to travel through the device layer, leaving a large number of defects in their track, thus degrading the material. While the issue might be circumvented by regrowth of pristine material [29] , quality factors of ion-irradiation-fabricated membranes have so far been limited to Q ≲ 20,000 (ref. 30) [30] . In this contribution, we report on two significant advances made towards ultrasensitive diamond nanomechanical resonators. In the first part, we present two strategies to fabricate high-quality and high-aspect ratio (>2,000:1) nanocantilevers from ultrapure, single-crystalline diamond starting material, achieving a processing level comparable to silicon. In the second part, we show that these procedures lead to nanomechanical resonators with exceptional quality factors ( Q >10 6 ) and low-intrinsic dissipation. Finally, we gain significant insight into the underlying physical dissipation mechanisms that provide rational basis and strategies for further improvement of diamond MEMS and NEMS. Device fabrication The basic fabrication pathway is shown in Fig. 1 . Our route taken starts with mm-sized single-crystal diamond plates of 20–40 μm thickness and <100> surface orientation grown by chemical vapour deposition [25] . The advantage of these plates is the high material quality (single crystal, low doping) and the fact that they are commercially available. The large thickness variation (up to 10 μm over the entire plate) and the delicate handling, however, are significant obstacles if large-area, sub-micron-structures are to be made. We have therefore developed a template-assisted repolishing procedure to improve thickness uniformity to <1 μm based on a polycrystalline diamond mould. To facilitate handling, we have implemented two different bonding strategies: In the first approach, we achieved direct wafer bonding to a thermal oxide-bearing silicon substrate using hydrogen silsesquioxane (HSQ) resist as intermediary. The advantage of this approach is a generic diamond-on-insulator (DOI) substrate amenable to any type of follow-up lithography. In the second strategy, we have clamped diamond plates between two SiO 2 substrates resulting in a fused ‘quartz sandwich’ structure. The advantage of this method is the simpler and faster processing exploiting quartz as both the handling substrate and mask material. In the next step, the diamond device layer was thinned to <500 nm using reactive ion etching based on an argon–chlorine (Ar/Cl) plasma [31] . This procedure is known to produce very uniform and smooth etches with resulting surface roughness well below 1 nm–rms. Cantilevers were then defined by standard optical lithography before they were fully released by backside etching steps. For samples made with the quartz sandwich method, a thick diamond ledge (~5 μm) was conserved at the base of the cantilevers to reduce clamping losses, while for DOI devices, the SiO 2 layer served as the clamping structure. Despite these precautions, clamping loss was observed in overetched DOI and some of the short sandwich devices (see Supplementary Figs 1–3 ). Micrographs of several devices are shown in Fig. 1h–j . More details on device fabrication are given in the Methods section. 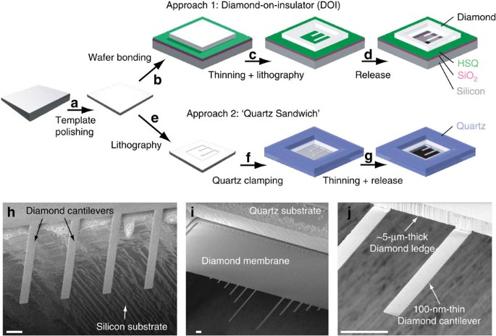Figure 1: Batch fabrication of single-crystal diamond nanocantilevers. (a) A roughly 3 × 3 × 0.03 mm3single-crystal diamond plate is template-polished to a thickness uniformity <1 μm over the entire plate. (b) In the DOI approach, the plate is first wafer bonded using HSQ to form a DOI substrate. (c) Plate is thinned to 0.1–1 μm thickness by reactive ion etching, and cantilevers are patterned using optical lithography. (d) Cantilevers are released using conventional backside etching. (e) In the ‘quartz sandwich’ approach, cantilevers are first patterned using optical lithography. (f) Diamond plate is clamped between two fused quartz slides with an ~2 × 2 mm2central aperture. (g) Exposed diamond plate is etched down until cantilevers become released. (h) Scanning electron micrograph of finished DOI devices. (i,j) Scanning electron micrographs of finished ‘quartz sandwich’ devices. Scale bars are 20 μm. Figure 1: Batch fabrication of single-crystal diamond nanocantilevers. ( a ) A roughly 3 × 3 × 0.03 mm 3 single-crystal diamond plate is template-polished to a thickness uniformity <1 μm over the entire plate. ( b ) In the DOI approach, the plate is first wafer bonded using HSQ to form a DOI substrate. ( c ) Plate is thinned to 0.1–1 μm thickness by reactive ion etching, and cantilevers are patterned using optical lithography. ( d ) Cantilevers are released using conventional backside etching. ( e ) In the ‘quartz sandwich’ approach, cantilevers are first patterned using optical lithography. ( f ) Diamond plate is clamped between two fused quartz slides with an ~2 × 2 mm 2 central aperture. ( g ) Exposed diamond plate is etched down until cantilevers become released. ( h ) Scanning electron micrograph of finished DOI devices. ( i , j ) Scanning electron micrographs of finished ‘quartz sandwich’ devices. Scale bars are 20 μm. Full size image For the present study, we have fabricated four single-crystal diamond chips bearing roughly ~25 cantilevers each. Three devices were made using the quartz sandwich method and one using the DOI method. We found both methods to be highly robust, achieving an overall 106 out 108 cantilever yield. Of the four devices, three were fabricated from ‘optical-grade’ starting material (Delaware Diamond Knives Inc.) with a doping concentration [ N ] <1 p.p.m., and a fourth chip was made from ‘electronic-grade’ material (ElementSix) with a much lower doping of [ N ] <5 p.p.b., [ B ] <1p.p.b. Cantilevers were between 20 and 240 μm long, between 8 and 16 μm wide and between 80 and 800 nm thick. Thickness variation along the entire length was found to be less than 100 nm, even for the longest 240-μm-cantilevers. Corresponding resonance frequencies were between ω c /(2π)=2 kHz–6 MHz and spring constants were between k c =60 μN m −1 –300 N m −1 . In the following study, we concentrated on the thinnest and longest (highest aspect ratio) devices, as they are the most interesting for force sensing. Moreover, thermoelastic damping and clamping losses are negligible for these structures [12] , [32] . The large number of finished devices allowed us to obtain a detailed picture of the mechanical dissipation in these structures. In particular, we have assessed the dependence of the quality factor on geometry, surface termination, temperature and doping concentration. For these measurements, we used a custom-built force microscope apparatus operated under high vacuum (<10 −6 mbar) mounted at the bottom of a dilution refrigerator (80 mK–300 K). The high vacuum eliminated viscous (air) damping and the refrigerator both served for temperature-dependence studies and for minimizing thermomechanical noise. Quality factors Q were measured by the ring-down method using a low-power (≤10 nW) fibre-optic interferometer for motion detection [11] , [12] . More details on the experimental setup are provided in the Methods section. Quality factors between 4 and 300 K In a first set of experiments, we have measured the temperature-dependent quality factors between 3 and 300 K of nine diamond resonators in total. Two representative measurements, one of an electronic grade (low doping) and one of an optical-grade (high doping) device, are shown in Fig. 2a . A third and fourth curve of a polycrystalline diamond cantilever and an ultrasensitive single-crystal silicon cantilever are added for reference. The polycrystalline cantilever was produced from a 3–5 nm grain size material (Advanced Diamond Technology), while the silicon cantilever was identical to those used in single-spin detection experiments [3] , [11] and served as a ‘best-of-its-kind’ benchmark device. We have measured several additional diamond curves (see Supplementary Figs 4 and 5 ) and while there is some variability between resonators, we found the general features visible in Fig. 2a to reproduce well between replicates and fabrication methods. 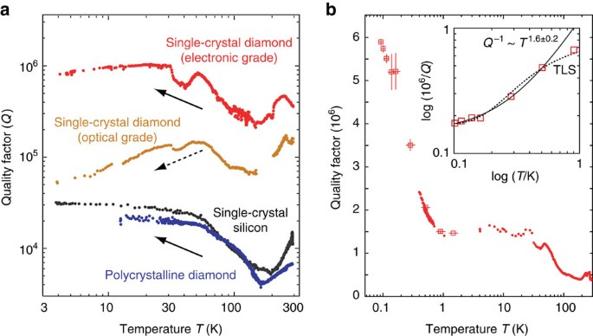Figure 2: Quality factors of single-crystal diamond nanoresonators between 0.1 and 300 K. (a) Two representative diamond devices (out of nine measured) are compared with refererence devices made from polycrystalline diamond and single-crystal silicon of similar thickness (100–300 nm).Qfactors between 100,000–1,000,000 are observed for diamond devices at room temperature, roughly 10–100 × higher than the reference devices. Cooling to 3 K leads to an increase inQfor the electronic grade (low doping) as well as the two reference resonators that are dominated by surface friction (solid arrows). Conversely, a reduction is seen inQfor the optical-grade (high doping) diamond resonator that has a strong contribution of bulk friction (dashed arrow). Single-crystal diamond devices were made by ‘quartz sandwich’ method and all diamond cantilevers were oxygen terminated. Silicon cantilever was according to ref.11. (b) Quality factor of a 660-nm-thick electronic-grade resonator in the millikelvin regime. Red dot data are obtained by sweeping refrigerator temperature, and red square data (with error bars) are obtained by varying the laser power incident at the resonator (see Methods). Solid black line is a power law fit withQ−1∝T1.6±0.2. Inset shows the 0.1–1 K data in a log-log plot against the standard tunneling model (solid line) and a model of thermally-activated two-level systems (TLS, dashed line). Additional parameters for all cantilevers can be found inTable 1. Figure 2: Quality factors of single-crystal diamond nanoresonators between 0.1 and 300 K. ( a ) Two representative diamond devices (out of nine measured) are compared with refererence devices made from polycrystalline diamond and single-crystal silicon of similar thickness (100–300 nm). Q factors between 100,000–1,000,000 are observed for diamond devices at room temperature, roughly 10–100 × higher than the reference devices. Cooling to 3 K leads to an increase in Q for the electronic grade (low doping) as well as the two reference resonators that are dominated by surface friction (solid arrows). Conversely, a reduction is seen in Q for the optical-grade (high doping) diamond resonator that has a strong contribution of bulk friction (dashed arrow). Single-crystal diamond devices were made by ‘quartz sandwich’ method and all diamond cantilevers were oxygen terminated. Silicon cantilever was according to ref. 11 . ( b ) Quality factor of a 660-nm-thick electronic-grade resonator in the millikelvin regime. Red dot data are obtained by sweeping refrigerator temperature, and red square data (with error bars) are obtained by varying the laser power incident at the resonator (see Methods). Solid black line is a power law fit with Q −1 ∝ T 1.6±0.2 . Inset shows the 0.1–1 K data in a log-log plot against the standard tunneling model (solid line) and a model of thermally-activated two-level systems (TLS, dashed line). Additional parameters for all cantilevers can be found in Table 1 . Full size image Figure 2a immediately reveals several interesting features. First, and most strikingly, we observe that single-crystal diamond resonators show very high-quality factors. For instance, the room temperature Q values of the two diamond resonators shown are 150,000 and 380,000 with a device thickness of only 100 nm and 280 nm, respectively (see Table 1 ). Other resonators showed room temperature Q factors up to 1.2 million at a thickness of 800 nm (see below). These values are between one and two orders of magnitude higher than similar polycrystalline [27] and single-crystal silicon resonators [12] , [13] . Table 1 Mechanical properties for selected cantilevers. Full size table Second, Fig. 2a shows a clear difference between the electronic-grade (low doping) and optical-grade (high doping) single-crystal diamond resonators. Most prominently, we observe that the Q factor of the electronic-grade resonator (and the two reference devices) increases towards cryogenic temperatures, while that of the optical-grade resonator decreases. Our understanding of this difference is as follows (more evidence will be given below): at room temperature, mechanical dissipation of all resonators is limited by surface friction. Surface friction is the most common dissipation mechanism for submicron-thick cantilevers [12] , [13] and commonly attributed to surface passivation layers or adsorbate molecules. Because devices show a similar behaviour as they are cooled from 300 K, the surface dissipation mechanism appears generic, such as related to common adsorbates. As temperatures approach 3 K, surface friction is markedly reduced (reflected in higher Q values) but it remains the dominating dissipation mechanism. The only exception is the optical-grade resonator: Here, a second friction mechanism begins to dominate at 3 K, reflected in lower Q values. As the only nominal difference between the electronic- and optical-grade diamond resonators is their doping concentration, it would be natural to assume that bulk impurities are related to the increase in friction. Quality factors at millikelvin temperatures To explore the potential of diamond nanomechanical resonators for millikelvin applications [3] , [8] , we have investigated dissipation in the best electronic-grade resonator down to about 0.1 K. These data are shown in Fig. 2b . We find that below about one kelvin, the Q factor further increases and for this particular device attains a value of almost six million at base temperature (~93 mK). This is the highest Q factor we have observed in this study. We have assessed four additional electronic-grade resonators at refrigerator base temperature (~400 mK resonator temperature, see Methods), and found that while some devices do show an increase in Q compared with 4 K, others do not (see Supplementary Table 1 ). We have seen a similar variability already with the (large dataset) of optical-grade devices in the 4–300 K-range, and attribute it to the fact that single-crystal diamond often has growth sectors of different quality even in the same crystal [33] and to variability in device fabrication. The manifestation of high Q factors at millikelvin temperatures, even if not observed in all devices, underlines that diamond as a material—if of high quality—has very low-intrinsic dissipation. We have attempted to explain the low-temperature increase in Q based on the standard tunnelling model [32] , [34] . For this purpose, we have fit the millikelvin data to a power law as , yielding a baseline quality factor of Q 0 =6.8·10 6 and T 0 =0.3 K. The exponent ε =1.6±0.2 is, however, considerably larger than the ε =0.5 predicted by the standard tunnelling model, indicating that the model does not fully describe the dissipation in our nanoresonators at low temperatures. We have found that the data fits reasonably well to a thermally-activated model that assumes an ensemble of identical two-level systems (TLS) non-resonantly coupled to the resonator mode (see Supplementary Note 1 ). In the TLS model, the baseline quality factor is Q 0 =5.9·10 6 and the thermal activation barrier is Δ E/h ~13 GHz. Both the power law and TLS models are plotted in the inset to Fig. 2b . Surface termination To further investigate the dissipation mechanism, we have surveyed between 15 and 40 optical-grade resonators under three different chemical surface terminations. This second set of measurements served to explore whether surface chemistry affects dissipation, and to find out whether diamond resonators can be improved by proper choice of surface termination. In the first round, cantilevers were measured ‘as-released’ right after the final Ar/Cl plasma reactive ion etch. In this state, the surface has a mixture of covalently attached elements, including H, O and Cl (see atomistic sketch in Fig. 3 ). In the second round, the surface was oxygen terminated using low-temperature (450 °C ) annealing in air [35] . O-termination represents the standard hydrophilic surface termination of diamond [36] . In the third round, the oxygen termination was converted to fluorine termination using CF 4 plasma [37] . F-termination is known to produce a simple monolayer coverage that is both hydrophobic and oleophobic with little molecular adsorption. We found O-terminated cantilevers to be very stable with no measurable degradation in Q after a two-months exposure to ambient atmosphere (F-terminated cantilevers were not remeasured). 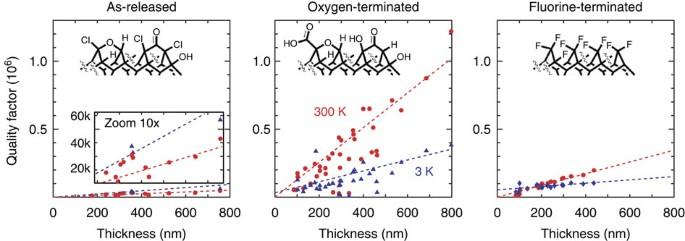Figure 3: Impact of surface chemistry on dissipation. Three different chemical surface terminations (sketched) are investigated on 15–40 devices of an optical-grade chip. Red dots are 300 K values and blue triangle are 3 K values, and dashed lines serve as guides to the eye. Large variation ofQfactors is seen as surface chemistry and thickness are changed, underlining the critical role of surface friction. Very highQfactors, exceeding one million at room temperature, are found for oxygen-terminated devices. Figure 3: Impact of surface chemistry on dissipation. Three different chemical surface terminations (sketched) are investigated on 15–40 devices of an optical-grade chip. Red dots are 300 K values and blue triangle are 3 K values, and dashed lines serve as guides to the eye. Large variation of Q factors is seen as surface chemistry and thickness are changed, underlining the critical role of surface friction. Very high Q factors, exceeding one million at room temperature, are found for oxygen-terminated devices. Full size image The data of these measurements are shown in Fig. 3 and are grouped by surface termination. We immediately see that the particular surface chemistry has a strong impact on dissipation, with more than 10-fold variation between ‘as-released’ and O-terminated devices. While the improvement with O- and F-termination compared with the ‘as-released’ state can be understood in terms of cleaner surfaces with better-defined surface chemistries (see Methods), the superior performance of O-terminated compared with F-terminated devices poses more challenges to interpretation. One hypothesis is that the terminating atoms are directly responsible for dissipation with little influence of adsorbates, and that F-atoms more efficiently engage in energy relaxation. Another hypothesis is that the inductive withdrawing effect of the polar C–F chemical bonds stabilizes a layer of electronic defects right below the surface that enhances energy relaxation [38] . If the second interpretation were true, it would be interesting to examine less polar termination groups including chlorine, sulphur, amine, hydrogen and alkyl groups [39] . Besides the variation with surface chemistry, we also observe that most plots in Fig. 3a–c show a roughly linear relationship between Q and thickness (shown by dashed lines). A thickness dependence of Q indicates a surface-related dissipation mechanism, whereas no thickness dependence would be characteristic of a bulk friction mechanism. The linear relationship between Q and thickness is most pronounced at 300 K (red data); at 3 K (blue data), the linear dependence is much weaker and Q values between O-terminated and F-terminated resonators converge. These observations confirm the picture from the temperature-dependence study in Fig. 2a : at room temperature, all resonators are limited by surface friction independent of surface chemistry, while at 3 K, bulk friction is strongly contributing and mostly dominating for F-terminated devices. In an attempt to compare presented diamond resonators to existing devices made from silicon or polycrystalline diamond, we have compiled a number of Q values from the literature and plotted them alongside the single-crystal diamond data from Fig. 3 . The comparison is shown in Fig. 4a . We find that for the same device thickness, single-crystal diamond may offer between one and two orders of magnitude higher Q factors compared with silicon or polycrystalline diamond. To make a similar comparison representative for force-sensing applications, we must also take material stiffness and density into account, which affect sensitivity through k c and f c (see Equation (2)). Assuming that Q is limited by surface dissipation and thus scales linearly with thickness, Equation (2) can be rewritten as , where w is a cantilever’s width, t its thickness, and l its length (see Supplementary Note 2 ). 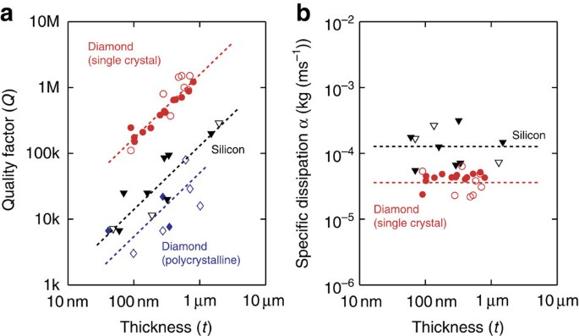Figure 4: Comparison ofQfactors between nanomechanical resonators made from different materials. (a) Comparison ofQfactors highlighting that for similar device dimensions, quality factors of single-crystal diamond are consistently higher by about an order of magnitude over single-crystal silicon devices. (b) Comparison of the geometry-independent dissipation parameter α (see Equation 3). Open symbols are 300 K values and filled symbols are ~4 K values. Dashed lines indicate linear thickness dependence ofQ. Data sources: single-crystal diamond data are from this study. Silicon ~4 K data are from ref.12and references therein. Silicon 300 K data are from a ~1.3 μm-thick cantilever withQ~380,000 (Nanoworld, Arrow TL1Au), a ~70 nm thick cantilever withQ~8,200 (custom-made), and the 135 nm-thick silicon reference cantilever withQ~11,000 (Table 1). Polycrystalline diamond cantilever data are from refs27,49,50,51. Figure 4: Comparison of Q factors between nanomechanical resonators made from different materials. ( a ) Comparison of Q factors highlighting that for similar device dimensions, quality factors of single-crystal diamond are consistently higher by about an order of magnitude over single-crystal silicon devices. ( b ) Comparison of the geometry-independent dissipation parameter α (see Equation 3). Open symbols are 300 K values and filled symbols are ~4 K values. Dashed lines indicate linear thickness dependence of Q . Data sources: single-crystal diamond data are from this study. Silicon ~4 K data are from ref. 12 and references therein. Silicon 300 K data are from a ~1.3 μm-thick cantilever with Q ~380,000 (Nanoworld, Arrow TL1Au), a ~70 nm thick cantilever with Q ~8,200 (custom-made), and the 135 nm-thick silicon reference cantilever with Q ~11,000 ( Table 1 ). Polycrystalline diamond cantilever data are from refs 27 , 49 , 50 , 51 . Full size image is a specific mechanical dissipation parameter that is now independent of geometry, yet contains all material properties. We note that α is related to the (geometry-dependent) ‘loss parameter’ γ = k c /( Q ω c ) [12] by γ ∝ α ( wt 2 / l ). Values for α are plotted in Fig. 4b . The plot confirms that diamond shows consistent low dissipation, although the improvement compared to silicon is somewhat less than with the mechanical Q due to the increased stiffness and density of diamond. It is furthermore instructive to evaluate the mechanical dissipation levels of diamond in the light of applications in quantum nanomechanics or ultrasensitive force sensing. Although our low-frequency resonators have a mean quantum mechanical occupation number that is far from the quantum mechanical ground state, we notice that their thermal decoherence time is quite long. For the device shown in Fig. 2b , for example, we find and τ≈ 0.5 ms at T =93 mK. This thermal decoherence time is long and well exceeds the oscillation period of T c =1/ f c ≈30 μs. could be reduced, for example, by going to lower temperatures [40] or by active feedback cooling [41] . could also be reduced by going to higher-frequency geometries [42] , although it remains to be seen if the high Q factors are maintained at much higher frequencies. The exciting prospect of presented resonators is that the low mechanical dissipation may be combined with other virtues of the diamond host material, such as optical transparency and high-quality nitrogen-vacancy impurities. Current resonators may be especially suitable for hybrid quantum architectures that do not a priori need ground state cooling, such as quantum spin transducers based on nanoelectromechanical resonator arrays [43] . We have also assessed the sensitivity of these resonators toward the measurement of small forces. The force sensitivity achievable by a freely vibrating resonator is ultimately limited by its thermal motion, equivalent to a thermal force noise F th given through Equation (2). According to the equipartition theorem, a mechanical force sensor is thermally limited if its noise temperature equals , where x rms is the rms displacement. We have analysed x rms by integrating the displacement spectral density in the vicinity of the cantilever resonance (see Methods and Supplementary Fig. 8 ), and found it to be in agreement with the predicted thermal motion down to about 10 K (depending on the particular device), but to be inaccurate below 10 K due to slight mechanical disturbance by the refrigerator circuit. Below 10 K, we have therefore inferred T using a combination of different bath temperatures and interferometer laser intensities, as explained with Fig. 2b . Using known values of k c , ω c , Q and T , we can then calculate the thermal force noise F th according to Equation (2). For the cantilever shown in Fig. 2b , we find F th =0.11fN Hz −1/2 at room temperature, 6aN Hz −1/2 at 3 K, and 0.54aN Hz −1/2 at 100 mK (see Table 1 . Other cantilevers in this study had a thermal force noise as low as 26aN Hz −1/2 at room temperature and 3.5aN Hz −1/2 at 3 K. These values are remarkable considering that the geometry of these test devices is not particularly optimized. With the present diamond material and processing method, we are confident that a cantilever thickness as small as 50 nm and a width of 1 μm could be realized for a 240-μm-long cantilever. Such a cantilever has a projected thermal force noise of 9.4aN Hz −1/2 at 300 K, 0.49aN Hz −1/2 at 3 K and 45zN Hz −1/2 at 100 mK, based on the scaling of F th with geometry (see Supplementary Note 2 ) and the Q ∝ t scaling of the quality factor. In conclusion, we have presented measurements of mechanical dissipation in submicron-thick single-crystal diamond nanomechanical resonators. We find that single-crystal diamond is an excellent material for mechanically resonant structures, with Q factors that are between one and two orders of magnitude higher than corresponding polycrystalline diamond devices, and one order of magnitude higher than similar silicon resonators. Measurements of the Q factor at room and cryogenic temperatures furthermore underline the importance of both surface quality and low-defect bulk material. Several possible avenues for reducing dissipation exist in both departments, including different surface chemistries [39] , atomic surface flatness [44] , reduction of intrinsic defects through high-temperature annealing [45] , or even the use of isotopically pure diamond material [46] . Moreover, we expect that geometry can be significantly optimized without unduly compromising device yields, moving thermally limited force sensitivities from the current ~0.54aN Hz −1/2 into the 10–100zN Hz −1/2 -range. Beside the demonstrated high mechanical quality factors and low mechanical dissipation, we believe that broad applicability of reported fabrication methods is a second main advance presented here. The facile and robust wafer bonding approaches result in general DOI or quartz-bonded substrates that are amenable to essentially any type of follow-up lithography. Due to its low absorption and high refractive index, for example, high-quality single-crystal diamond would be ideally suited for use in optomechanical cavities or as photonic crystal material [47] . Diamond further possesses interesting lattice defects, such as nitrogen-vacancy centres, that could be directly embedded in high- Q diamond NEMS and enable direct coupling between mechanical, spin and optical degrees of freedom [9] , [48] . Such on-chip devices are considered key components for hybrid quantum systems in quantum science and technology, underscoring the prominent material platform diamond can offer to future applications. Device fabrication Diamond material and polishing: Diamond plates were purchased from ElementSix and Delaware Diamond Knives (DDK). Dimensions were roughly 3 × 3 mm 2 laterally and 20–40 μm in thickness, with a typical wedge of 5–15 μm over the entire plate. Plates were laser cut to size and had a surface polish of <5 nm. Both surfaces were briefly plasma etched to remove the first ~100 nm on each side to improve surface quality. Surface roughness after etching was not measured on these samples but was ≤0.4 nm–rms over a 300 × 300 nm 2 area for an equivalent sample in a different study. Wedged plates were repolished by placing them in a custom-made polycrystalline diamond mould of ~20 μm depth, resulting in an improvement of surface unformity better than 1 μm. All plates had a <100> surface orientation. Electronic-grade plates (ElementSix) had a doping concentration of and <5 p.p.b. [B]. Optical-grade plates (DDK) had a doping concentration of and <5 p.p.m. [B]. DOI wafer bonding: both the diamond and the handling substrate were cleaned for 10 min in a boiling piranha solution and rinsed with deionized water. Diamond was allowed to dry in air, placed on a clean room wipe, whereas the handling substrate was blown dry with nitrogen. After a 10-min dehydration bake of both pieces at 200 °C in air, HSQ resist was spin-coated onto the handling chip at 2,000 r.p.m. for 10 s. The diamond plate was quickly placed on top of the freshly spun HSQ layer, with its originally upward-facing surface making contact with HSQ. The assembly was annealed under a uniform pressure of 10 5 kPa at 500 °C for 30 min. Quartz sandwich wafer bonding: to sandwich the diamond between quartz slides, both quartz slides were cleaned in boiling piranha solution. Both slides had through holes in the centre for access to the diamond membrane. One of them had a an additional 20-μm-deep pit patterned at the centre to accommodate the ~20 μm-thick diamond plate and to allow for direct contact between the quartz slides. Bonding was achieved using a uniform pressure of 10 5 kPa at 500 °C for 30 min. Cantilever patterning and release: cantilever patterns were defined using oxygen-based plasmas using plasma-enhanced chemical vapour deposition oxide as the hardmask. Silicon wafer through etch was performed using a standard Bosch process, with a 10-μm-positive photoresist. Release from the silicon oxide etch-stop membrane was performed in buffered hydrofluoric acid (HF), followed by copious rinsing in deionized water and isopropyl alcohol. The cantilever chip was directly retracted from the isopropyl alcohol and allowed to dry in air. The progress of diamond thinning by Ar/Cl 2 inductively coupled plasma in the DOI approach was monitored by profilometry. The progress of diamond thinning and concurrent cantilever release by the same plasma in the sandwich method was monitored using thin-film ellipsometry. Surface modification: In the ‘as-released’ state, the surface had a mixture of covalently attached H, O and Cl, as confirmed by X-ray photoelectron spectroscopy measurements. Moreover, SiO 2 particles were sometimes found to be present, as SiO 2 from the mask can redeposit during plasma etching. Possible SiO 2 was later removed using an additional HF cleaning step. HF cleaning lead to a slight (2 × ) improvement of Q factors, but nowhere close to the Q factors found for O-terminated or F-terminated devices.Oxygen termination of the diamond surface was achieved by a low-temperature (450 C) annealing in air [35] . The air annealing step has the added benefit of removing organic and graphitic contamination from the surface leading to a general improvement of surface quality. Fluorine termination was achieved using exposure to a CF 4 plasma [37] . Polycrystalline diamond cantilevers: polycrystalline diamond reference cantilevers were produced from ultrananocrystalline (3–5 nm grain size) material, available as a DOI wafer from Advanced Diamond Technology, using applicable steps from our DOI method. Experimental setup Mechanical properties of diamond nanoresonators were measured in a custom-built scanning force microscope designed for magnetic resonance force microscopy [3] . Cantilevers were prepared under ambient conditions and then mounted in a high-vacuum chamber (<10 −6 mbar) at the bottom of a dilution refrigerator (~80 mK–300 K). Resonator frequency ω c and quality factor Q were measured using the ring-down method [12] , and the spring constant k c calibrated via a thermomechanical noise measurement at room temperature [11] . As a consistency check, ω c and k c were independently calculated from the geometry using a finite element software (COMSOL). Resonator motion was detected using a low-power fibre-optic interferometer operating at a wavelength of 830 nm and producing less than 10 nW of laser light incident at the cantilever. To exclude cavity effects, it was verified that the same Q factor was obtained whether the measurement was done on the positive or negative (red- or blue-shifted) side of the interferometer fringe. Variable temperature measurements To measure temperature dependence of quality factors, two complementary measurement techniques were employed. For temperatures between 0.4–300 K, Q ( T ) was measured the usual way by slowly ( ≲ 0.2 K min −1 ) sweeping refrigerator temperature and assuming thermal equilibrium between resonator and bath. For very low temperatures ( T <2K), the refrigerator was operated at base temperature (80 mK) and resonator temperature was adjusted by varying interferometer laser power through absorptive heating (see Supplementary Note 3 ). The advantage of the latter method is that resonator temperature can be directly estimated via the low-temperature thermal conductivity of diamond. (Cantilever mode temperature could also be inferred from a thermomechanical noise measurement [11] , but this method was inaccurate <10 K due to slight mechanical vibrations introduced by the refrigerator circuit.) Further details are given in Supplementary Notes 3 and 4 . How to cite this article : Tao, Y. et al. Single-crystal diamond nanomechanical resonators with quality factors exceeding one million. Nat. Commun. 5:3638 doi: 10.1038/ncomms4638 (2014).